Regeneration limit of classical Shannon capacity Since Shannon derived the seminal formula for the capacity of the additive linear white Gaussian noise channel, it has commonly been interpreted as the ultimate limit of error-free information transmission rate. However, the capacity above the corresponding linear channel limit can be achieved when noise is suppressed using nonlinear elements; that is, the regenerative function not available in linear systems. Regeneration is a fundamental concept that extends from biology to optical communications. All-optical regeneration of coherent signal has attracted particular attention. Surprisingly, the quantitative impact of regeneration on the Shannon capacity has remained unstudied. Here we propose a new method of designing regenerative transmission systems with capacity that is higher than the corresponding linear channel, and illustrate it by proposing application of the Fourier transform for efficient regeneration of multilevel multidimensional signals. The regenerative Shannon limit—the upper bound of regeneration efficiency—is derived. Shannon capacity [1] defines the maximum amount of error-free information that can be transmitted through a communication channel. Although the linear Shannon limit [1] was calculated in 1948, there is no unique nonlinear Shannon limit, as nonlinearity can occur and can be designed and modified in various ways. However, the current existing estimations for lower bounds [2] , [3] , [4] , [5] on the Shannon capacity are still referenced as the nonlinear Shannon limit. The calculation of the Shannon capacity for different nonlinear channels is an open and challenging problem. The existing optical communication systems and technologies, which are primarily responsible for the global data traffic, are facing serious challenges due to nonlinear properties of fibre channels [2] , [3] , [4] , [5] . It is fair to say that the optical communication sector has reached a bifurcation point and a number of fundamentally new methods to improve information transmission are under investigation around the world (see, for example, refs 6 , 7 , 8 and references therein). All-optical regeneration, being energy efficient and effective mitigation of noise impairments, attracts attention as a powerful tool for improving quality of signal transmission [9] , [10] , [11] , [12] , [13] , [14] , [15] , [16] , [17] , [18] , [19] . In the current study, we develop a theoretical framework for calculating the Shannon capacity (mutual information optimized over input signal distribution, as defined by Shannon) for nonlinear regenerative channels illustrating it on the example of the proposed regenerative Fourier transform (RFT). Moreover, the maximum gain in Shannon capacity due to regeneration (that is, the Shannon capacity of a system with ideal regenerators—the upper bound on all regenerative schemes) is calculated analytically; thus, the regenerative limit to which the capacity of any regenerative system can be compared, as analogue of the seminal linear Shannon limit, is derived for constructive nonlinearity. Regenerative mapping We propose a new technique—the regenerative mapping (see Fig. 1a,b )—for designing the classes of nonlinear communication channels with capacity exceeding the Shannon capacity of the linear additive white Gaussian noise (AWGN) channel. An important new feature introduced by the considered nonlinear mapping is the potential for continuous nonlinear filtering with signal regeneration without requiring a hard decision. This differs from traditional approaches based on ideal regenerators [19] , which are characterized by step-like piecewise transfer function. The proposed practical example of regenerative mapping incorporates experimentally verified regenerative models [12] , [20] and enables analytical optimization. Whenever the nonlinear transformation has multiple fixed points ( Fig. 1c ), the consequent interleaving of the accumulating noise with the nonlinear filter produces effective suppression of the noise (see Fig. 1d ). The created washboard potential ( Fig. 1c ) quantizes the signal and improves transmission, with a consequent increase in capacity. A similar idea has been discussed in multiple contexts, ranging from physical systems [21] to the interpretation of biological memory effects in terms of potentials with multiple minima [22] . In quantum theory, a qualitatively similar phenomenon is known as the Zeno effect, where continuous measurement of the quantum system and associated von Neumann collapse of wave function prevents the natural dispersion of the wave function and causes the quantum system to remain in the same state [23] . 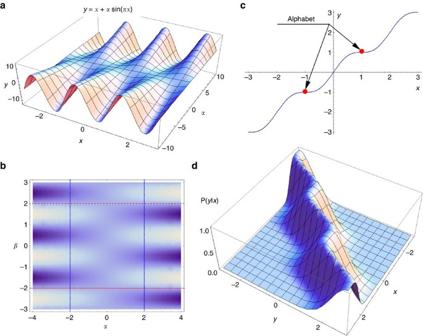Figure 1: The regenerative transfer function. y=T(x)=x+αsin(βx) (a) plotted with fixedβ=πshows periodic washboard potential with the slope defined by the parameters; (b) transfer function (TF) with varyingαandβatx=πhigher intensity is shown by a lighter colour, the optimal values are shown by dashed lines; (c)y=T(x) for the parametersβ=πandα=1/β—the optimal set of parameters defines zero slope at the stationary points (maximum noise suppression); (d) Gaussian conditional PDFP(y|x) for the channel with one filter with TF,y=x+π−1sin(πx) illustrates the regeneration effect at the points defining the signal alphabet. Figure 1: The regenerative transfer function. y = T ( x )= x + α sin( βx ) ( a ) plotted with fixed β = π shows periodic washboard potential with the slope defined by the parameters; ( b ) transfer function (TF) with varying α and β at x = π higher intensity is shown by a lighter colour, the optimal values are shown by dashed lines; ( c ) y = T ( x ) for the parameters β = π and α =1/ β —the optimal set of parameters defines zero slope at the stationary points (maximum noise suppression); ( d ) Gaussian conditional PDF P ( y | x ) for the channel with one filter with TF, y = x + π −1 sin( πx ) illustrates the regeneration effect at the points defining the signal alphabet. Full size image Consider a regenerative channel with R identical nonlinear filters placed along the transmission line. The cascaded regeneration was demonstrated for various regenerative schemes [16] , [17] , [18] . The signal transmission (for simplicity, signal propagation between the regenerators is assumed to be linear) is distorted by an AWGN that is uniformly distributed along the line, which can be considered as an analogue of the random force in the time-continuous case or noise mixing with the signal during transmission through the media. The regenerative map has a set of special points that are optimal for the nonlinear filtering. The nonlinear transformations y = T ( x ) (see Fig. 2 ) result in the effective potential, which creates attraction regions in the signal mapping. When the points are ‘attracted’ to the alphabet, the alphabet should remain stable. 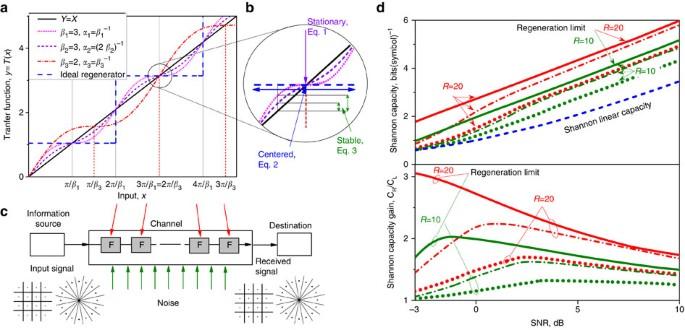Figure 2: The regenerative channel model. (a) The regenerative transfer functions, plotted for the ideal regenerator and RFT:y=x+αsin(βx) with the alphabet shown by vertical lines; (b) the graphical interpretation of the stability analysis; (c) the scheme with regenerative filters (denoted by F) placed equidistantly along the line; noise distortions are effectively filtered by the ideal regenerators (see constellations before and after noisy transmission with attraction regions shown by straight lines); and (d) numerically calculated Shannon capacity and gain (compared with the linear AWGN channel) for RFT channel withR=20 andR=10 filters (showed by red and green colours, respectively) for both the superstable (dashed-dotted)αβ=1 and stable (dotted)αβ=0.5 mapping. The upper bounds of regeneration efficiency for the given number of the ideal filtersR=10 andR=20 are shown by solid green and red curves, respectively. This leads to the following set of conditions imposed on the transfer function: Figure 2: The regenerative channel model. ( a ) The regenerative transfer functions, plotted for the ideal regenerator and RFT: y = x + α sin( βx ) with the alphabet shown by vertical lines; ( b ) the graphical interpretation of the stability analysis; ( c ) the scheme with regenerative filters (denoted by F) placed equidistantly along the line; noise distortions are effectively filtered by the ideal regenerators (see constellations before and after noisy transmission with attraction regions shown by straight lines); and ( d ) numerically calculated Shannon capacity and gain (compared with the linear AWGN channel) for RFT channel with R =20 and R =10 filters (showed by red and green colours, respectively) for both the superstable (dashed-dotted) αβ =1 and stable (dotted) αβ =0.5 mapping. The upper bounds of regeneration efficiency for the given number of the ideal filters R =10 and R =20 are shown by solid green and red curves, respectively. Full size image The first condition means that the alphabet is defined by the stationary points x * of the mapping. Next, the transfer function should change curvature at the alphabet; in other words, the alphabet point is the centre of the attraction region. The third expression reflects the stability condition; that is, the distortion of the signal points is effectively suppressed (see geometry in Fig. 2b ). When the first derivative is equal to zero, the alphabet is called superstable. Regenerative Fourier transform As an illustration, we propose the regenerative Fourier transform (RFT). The concept of RFT (see Supplementary Fig. 1 , Supplementary Note 1 ) may be generalized to any complete orthogonal system of functions. Without any loss of generality, we use sine functions as the basis for the expansion. The input signal is described by the waveform: , here summation is performed over the number of symbols, f ( t ) is a carrier pulse shape and T s is a symbol period. We apply RFT to each quadrature and add the original and transformed signals: Integrated optics-based realization makes FT practically available for numerous emerging applications in optics [24] , [25] , [26] , [27] , [28] , [29] . We show that FT can be used for efficient signal regeneration: RFT. Being the FT of the ideal regenerator, described by the stepwise transfer function, RFT represents the highest achievable regeneration efficiency and can be applied to multilevel multidimensional signals. The RFT mapping is shown in Fig. 2a . According to the previously described optimization procedure, in the considered example the alphabet is placed at the points π (2 k +1)/ β , where k ε Z , that are stable if and only if αβ ≤1. In particular, the system is superstable when αβ =1, this gives the optimum parameter values, whereas inequality defines the suboptimal parameters range. As indicated in ref. 30 , it is challenging to regenerate high-order constellations (higher than 32) using the conventional approach of regenerating phase and amplitude, as such constellations have tight phase packing due to energy efficiency requirements. Therefore, a new approach for regenerating separately the two signal quadratures will be required. The proposed RFT is the first scheme to operate on both quadratures and enable an infinite number of regenerative levels. In this sense, this scheme will also potentially enable regeneration of the conventional modulation formats (like, for example, rectangular quadrature amplitude modulation). Moreover, RFT enables the high regeneration efficiency without making a hard decision. The calculated corresponding Shannon capacity shows that such a channel can provide a capacity above the classical Shannon capacity of the linear AWGN channel. Shannon capacity The definition of the Shannon capacity for an arbitrary channel (in what follows, capacity C is per unit bandwidth) involves maximizing the mutual information functional [1] : over all valid input probability distributions P ( x ) subject to the power constraint ∬ D xP ( x )| x | 2 ≤ S . Here, the statistical properties of the channel are given by the conditional output–input probability density function (PDF) P ( y | x ). Shannon capacity (equation (4)) of the considered systems is a function of the signal-to-noise ratio (SNR), the number of nonlinear filters R and the parameters of nonlinear mapping. SNR is defined here as the ratio of the input signal power S to the noise added linearly to the signal during transmission at each node k =1,…, R : SNR= S / N , where the accumulated noise is given by N =Σ N k with k being a temporal [31] , [32] or spatial index. Note that in the nonlinear communication system the definition of the in-line SNR is a nontrivial issue, due to the mixing of signal with noise during propagation. The introduced SNR has the meaning of the signal-to-noise ratio in the respective linear system in the absence of nonlinear in-line elements. This enables the comparison between the performance of the considered system and the corresponding linear AWGN channel with the same noise level. Evidently, the effect of noise squeezing is enhanced as the number of regenerators/nonlinear filters increases (see Fig. 3 ). To quantify the overall effect, we studied the capacity of the source-destination transmission as a function of the SNR that incorporates the resulting power of all added noise at the source-destination link, which is fundamentally different from the decode-and-forward channel model. 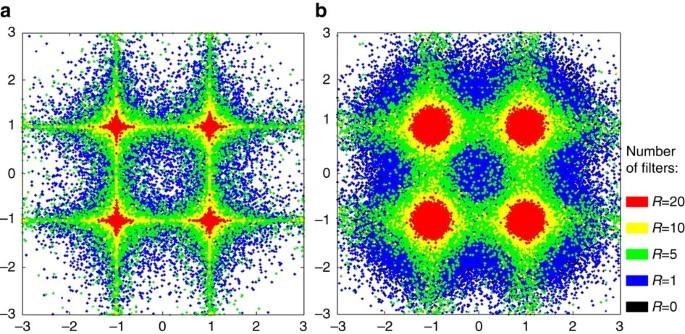Figure 3: Transmission improvement. RectangularM=4 constellations afterRconsequent RFT transformations interleaved with noise shown (a) at the output of theRth filter (after RFT transformation) and (b) at the receiving end (when the noise of the last span is added) for the transmission lines having fixed AWGN distortion of SNR=3 dB. The level of noise suppression is more pronounced for the higher number of in-line RFT filters characterized by TF:y=x+π−1sinπx. Linear unregenerated caseR=0 is shown for reference. Figure 3: Transmission improvement. Rectangular M =4 constellations after R consequent RFT transformations interleaved with noise shown ( a ) at the output of the R th filter (after RFT transformation) and ( b ) at the receiving end (when the noise of the last span is added) for the transmission lines having fixed AWGN distortion of SNR=3 dB. The level of noise suppression is more pronounced for the higher number of in-line RFT filters characterized by TF: y = x + π −1 sin π x. Linear unregenerated case R =0 is shown for reference. Full size image The numerically calculated Shannon capacity (mutual information optimized over all input PDF P ( x )) is shown in Fig. 2d , which demonstrates visible capacity gain over the Shannon capacity of the linear AWGN channel. In the limit of a large SNR and/or large number of nonlinear filters, all regenerative schemes tend towards asymptotic behaviour, when the gain gap between regenerative and linear AWGN channel capacity is constant. Using the method of steepest descent, we derive the capacity increase for the n -dimensional channel with the RFT transfer function for the suboptimal parameters’ relation (see equation (3)) q = αβ <1: Regenerative limit The capacity analysis of the system with the ideal regenerators defines the upper bound of regeneration efficiency. The ideal regenerators assign each transmitted symbol to the closest element of the given alphabet (the corresponding stepwise transfer function is plotted in Fig. 2a by the dashed blue line). At low SNR range, the Shannon capacity is well approximated by the following expression: with the transition matrix elements (denote SNR as ρ ): and m ± =1− m + . As the SNR increases, the distance between the closest neighbours reaches the optimal cell size, which is defined by the noise variance and the number of in-line regenerators, , with κ =1+10 R −1 and W is the so-called Lambert W function (further, we use normalized value ). Therefore, with the growing signal power, the amplitude distribution remains equidistant, whereas the maximum entropy principle defines Maxwell–Boltzmann distribution as the optimal PDF for a fixed average energy constraint (which is in agreement with performed numerical optimization). Thus, with the growing SNR, a constant gap (that quantifies improvement) can be seen between the regenerative channel and linear AWGN channel capacities (see Supplementary Note 2 ). The capacity improvement is defined by the noise variance and the number of regenerators: An additional noise induced from a device itself N T can be incorporated in equation (6), by substituting: N → N + RN T . Moreover, one can estimate a critical value for the noise variance, which can be squeezed by the transformation. By using regenerative mapping technique, it is possible to define a half-width Δ of a plateau (superstable choice of parameters: T ′( x *)=0) around an alphabet point x * by solving: T ′( x *+Δ)=1 (in particular, for RFT the condition defines: ). Therefore, the noise is reduced if N / R + N T ≤Δ. The maximum capacity gain due to regeneration (that is, the maximum regeneration efficiency) is observed for the binary channel. The capacity gain reflects the trade-off between the system complexity and capacity improvement. As the number of regenerators increases, the peak of the capacity gain shifts to a smaller SNR. Therefore, employing a low SNR regime and using regeneration, one can achieve high transmission performance with low energy consumption. The minimum SNR value, when d opt is achieved, defines the maximum capacity ratio to its linear analogue; that is, . At this SNR value, both analytic formulae equations (5) and (6) can be interpolated to describe capacity at the full range of the SNR. Numeric validation The analytical approximations shown by the black lines in Fig. 4a demonstrate an excellent agreement with the result of numerical computations of the Shannon capacity that exceeds the linear Shannon limit for different number of regenerators (here numerical optimization over input PDF was performed). 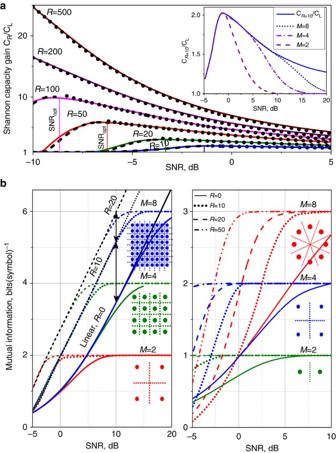Figure 4: Regeneration limit. (a) Gain, the regenerative Shannon capacity ratio to the Shannon formulaCL=log2(1+ρ), for the different number of regenerators. The analytical results shown by black (dashed) equation 5 and dotted using equation 6) lines demonstrate an excellent agreement with numerics (solid coloured lines). The inset shows mutual information gain forM2—rectangular constellations approaching capacity gain. (b) Capacity and mutual information for discreteM2—rectangular (left panel) andM—points in the ring (right panel) alphabets. The arrows show the constant capacity increase. Constellations and associated attraction regions are shown. Figure 4b shows the mutual information (here all symbols were assumed to be equiprobable) for rectangular (left panel) and ring (right panel) packing. Moreover, here we stress the importance of input signal optimization for capacity calculations in nonlinear regenerative channels; otherwise, nonlinearity (even constructive one) will degrade system capacity. Figure 4: Regeneration limit. ( a ) Gain, the regenerative Shannon capacity ratio to the Shannon formula C L =log 2 (1+ ρ ), for the different number of regenerators. The analytical results shown by black (dashed) equation 5 and dotted using equation 6) lines demonstrate an excellent agreement with numerics (solid coloured lines). The inset shows mutual information gain for M 2 —rectangular constellations approaching capacity gain. ( b ) Capacity and mutual information for discrete M 2 —rectangular (left panel) and M —points in the ring (right panel) alphabets. The arrows show the constant capacity increase. Constellations and associated attraction regions are shown. Full size image Note that the nonlinear regenerative channel is a fundamentally different (to linear AWGN channel) information channel with the constructive use of nonlinearity. In such nonlinear channels, the derived regenerative limit can be considered as the analogue of the Shannon linear limit—it is the maximum error-free transmission rate in regenerative channels. In fibre-optic channels, one can incorporate the impact of Kerr nonlinearity and dispersion on the channel capacity as first-order perturbation, whereas the main order is given by equations (5) and (6). The developed capacity calculation model can generally be applied to various regenerative schemes, where methodology (in Supplementary Note 3 , further illustrated on RFT Supplementary Note 4 ) can be adapted accordingly. The introduced class of regenerative channels has information capacity that exceeds the Shannon capacity of the linear AWGN channel. The gain is achieved by noise squeezing due to the introduced mapping filter that creates attraction regions around the stable alphabet. The model is generic and the obtained results can be applied to a wide range of physical problems. The results reveal a fascinating new aspect of the interplay between stochastic processes and system nonlinearity, stressing the impact on the channel capacity. The Shannon capacity is calculated by defining the conditional PDF, which is expressed through Onsager–Machlup functional or action of the path given by the stochastic map—a discrete version of the Langevin equation for the stochastic processes at each node (see Supplementary Note 3 ). The detailed description of the capacity functional optimization is given in the Supplementary Note 5 . How to cite this article: Sorokina, M. A. and Turitsyn, S. K. Regeneration limit of classical Shannon capacity. Nat. Commun. 5:3861 doi: 10.1038/ncomms4861 (2014).